Antipathogenic properties and applications of low-dimensional materials A major health concern of the 21 st century is the rise of multi-drug resistant pathogenic microbial species. Recent technological advancements have led to considerable opportunities for low-dimensional materials (LDMs) as potential next-generation antimicrobials. LDMs have demonstrated antimicrobial behaviour towards a variety of pathogenic bacterial and fungal cells, due to their unique physicochemical properties. This review provides a critical assessment of current LDMs that have exhibited antimicrobial behaviour and their mechanism of action. Future design considerations and constraints in deploying LDMs for antimicrobial applications are discussed. It is envisioned that this review will guide future design parameters for LDM-based antimicrobial applications. Antimicrobial agents play a vital role in the prevention of pathogenic bacterial and fungal infections, accounting for a predicted 95% reduction in mortality rates since their introduction in the late 1940s [1] , [2] , [3] , [4] . However, in recent times, over-prescription and misuse of antibiotics in medical, veterinary and agricultural industries, combined with the rapid evolution of microbial species, has contributed to the emergence of antimicrobial resistance (AMR) in pathogenic microbes [1] , [2] . Globally, single and multi-drug resistant (MDR) microbes are responsible for ~700,000 deaths each year [1] . The World Health Organisation (WHO), has named several concerning drug resistant, pathogenic bacterial strains prevalent in global healthcare settings, including MDR tuberculosis (MDR-TB), carbapenem-resistant Enterobacteriaceae (CRE), methicillin-resistant S taphylococcus aureus (MRSA) and MDR Neisseria gonorrhoeae [1] , [3] , [4] . Resistant fungal strains, including MDR Candida auris , are also becoming increasingly resistant to all available antifungal treatments [2] . Without the development of new antimicrobial agents, the WHO estimates that by 2050, approximately 10 million people will die annually from previously treatable infections [5] . The predicted economic impact of AMR suggests it could be worse than the 2008 global financial crisis [4] , costing over US$100 trillion in healthcare [5] . In response, considerable research has been conducted in an attempt to combat these infections [6] , [7] , [8] , [9] . Unfortunately, the development of new antimicrobial drugs has faltered in recent years, with only two new classes of antibiotics receiving approval from international regulatory agencies in the past 20 years [4] with neither being effective against Gram-negative bacteria. This has driven research towards the development of alternative antimicrobial nanomaterials including polymers [6] , particles [7] and surface coatings [8] . One of the first nanomaterials that demonstrated high antipathogenic abilities is silver nanoparticles and has subsequently received an extensive amount of attention in the research community [10] , [11] . More recently, low-dimensional materials (LDMs) have gained significant interest as potential antimicrobial agents [12] , [13] . These materials are categorised as zero-dimensional (0D) [14] , one-dimensional (1D) [15] or two-dimensional (2D) [16] nanomaterials based on their respective dimensionality. These materials have demonstrated favourable properties that have led to their use in electronics and sensing [17] , [18] . A more comprehensive understanding of the underlying properties of LDMs, in conjunction with improved fabrication methods has led to the development of LDMs for new applications, including biomedical [19] , [20] and antipathogenic technologies [15] , [21] . LDMs that have demonstrated antimicrobial activity across a range of dimensions include 0D black phosphorous (BP) [21] ; 1D zinc oxide (ZnO) [22] and 2D molybdenum disulphide (MoS 2 ) [23] ; among others [13] , [24] , [25] . The antimicrobial mechanisms of LDMs have not been clearly elucidated, and there remain conflicting opinions in the field, in part due to varied experimental designs and multifaceted antimicrobial mechanisms [26] , [27] . It is thought, however, that the antimicrobial activity can occur through both physical and chemical means, or in combination. Importantly, it has been suggested that LDMs can limit the potential development of microbial resistance, while also enabling control over the antipathogenic mechanisms through tuning the physico-chemical properties of the materials, such as size, shape and composition, including heterostructures and the addition of functional groups [13] , [28] . This review focuses on the current understanding of the antimicrobial mechanisms for LDMs and highlights areas which require further investigation. Initially, the antimicrobial mechanisms, including passive and stimuli-activated actions of LDMs, will be summarised. Following this, elemental and compound LDMs will be reviewed, focusing on graphene and graphene analogues, metal oxides (MOs), transition metal dichalcogenides (TMDs) and early transition metal carbides, nitrides and carbonitrides (MXenes) classes of materials. Finally, recent advancements in combined LDMs either as heterostructures or composite forms and their tunability in terms of antimicrobial activity will be analysed. The review concludes with a discussion of future design strategies for single and composite LDMs to optimise antimicrobial efficacy for next-generation treatments. LDMs can be classified as 0D, 1D, or 2D depending on their size and aspect ratios [29] . A visual summary of LDMs and their associated antimicrobial mechanisms are shown in Fig. 1 . 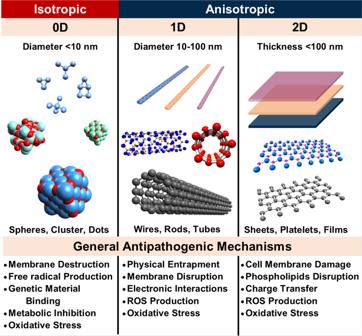Fig. 1: The contrast of 0D, 1D and 2D materials. Common structures for each dimensional classification and their general antimicrobial mechanisms. Some properties of common 0D, 1D and 2D materials are shown in Table 1 and their atomic structure and morphology are shown in Fig. 2 . Common LDMs include carbon, graphene (Gr), graphene oxide (GO), graphitic carbon nitride (g-C 3 N 4 ), BP, Boron nitride (BN), 2D hexagonal BN (hBN), MoS 2 , titanium carbide (Ti 3 C 2 T x ) MXene and MO such as ZnO, titanium oxide (TiO 2 ) and copper oxide (CuO). Fig. 1: The contrast of 0D, 1D and 2D materials. Common structures for each dimensional classification and their general antimicrobial mechanisms. Full size image Table 1 Properties of common LDMs. Full size table Fig. 2: Visual summary of common LDMs. 0D The chemical structure (top), high-resolution transmission electron microscope (HRTEM) image (inset is corresponding selected area electron diffraction (SAED) pattern where applicable) (middle) and atomic force microscopy (AFM) scan (bottom) for carbon dots [77] , [200] , BP QDs [201] , BN QDs [202] , g-C3N4 QDs [123] , MoS 2 NDs [168] , Ti 3 C 2 T x QDs [83] , ZnO QDs [133] , [203] and TiO 2 QDs [129] , [204] . 1D The chemical structure (top), HRTEM image (inset is corresponding SAED pattern) (middle) and AFM scan or scanning electron microscope (SEM) image (bottom) for carbon NWs [205] , BP NWs [18] , BN NFs [206] /NTs [207] , g-C 3 N 4 NRs [179] , [208] , MoS 2 NWs [91] , [209] , CuO NRs [86] , ZnO NWs [22] , [210] and TiO 2 NWs [12] /NTs [211] . 2D The chemical structure (top), HRTEM image (inset is corresponding SAED pattern) (middle) and AFM scan (bottom) for graphene (Gr) NSs [192] , GO NSs [212] , [213] , BP NSs [194] , hBN NSs [192] , g-C 3 N 4 NSs [214] , MoS 2 NSs [192] , Ti 3 C 2 T x NSs [43] , [215] and ZnO NSs [216] . Full size image 0D materials Zero-dimensional materials (0D materials) are confined to the nanoscale in all three dimensions and are composed of only a few atoms, resulting in an average size of less than 10 nm and uniform (i.e. isotropic) properties [30] . Quantum dots (QDs) are crystalline clusters of semiconductor materials [31] , while nanoclusters and nanodots (NDs) consist of a wider range of materials under 10 nm [30] , [32] . 0D materials have gained popularity due to their versatile size-dependent optical and physicochemical properties [14] , [30] , along with the possibility for biomedical applications, such as bioimaging [33] , [34] . Several advantages include tuneable oxidation potential [35] ; light-induced free radical generation [30] ; and high photothermal efficiency [14] . 1D materials One-dimensional (1D) materials are confined to the nanoscale in two dimensions while the remaining dimension is typically in the microscale. These materials form cylindrical structures with a diameter ranging from 10 to 100 nm and generally are less than 12 µm in length [12] , [15] . Nanorods (NRo) are characterised as solid structures with a low length to width aspect ratio in comparison to nanowires (NWs), nanotubes (NTs), nanoribbons (NRi) and nanofibers (NFs), which have a high length to width aspect ratios [36] , [37] . As the terms NWs and NFs are often used interchangeably, in this review, we classify NWs as structures composed of inorganic or metallic materials, whereas we define NFs as composed of organic materials [36] , [38] . NTs possess a hollow centre, typically with an internal diameter of under 100 nm and an external diameter up to 1 µm, which results in the highest surface area for 1D materials [37] . It should be noted that these NT dimensions are not absolute, and examples of larger materials being referred to at NTs in the literature are common. Unlike 0D materials, 1D materials are anisotropic as many of their physicochemical properties are non-uniformly distributed. Some favourable properties of 1D materials, include a larger/higher relative surface area, and tuneable oxidative stress and catalytic ability [22] , [36] , [39] . Within biological systems, 1D materials have been investigated for potential anticancer applications [40] and other biomedical application [41] , [42] . 2D materials Two-dimensional (2D) materials are only confined to the nanoscale in one dimension, and the other two dimensions typically span into the micro to centimetre scale [43] , [44] . They form nanosheets (NSs), also called nanoflakes, which can have more random shapes [45] . When materials have a more uniform and controlled configuration with straight edges, they are called nanoplatelets (NPs), or nanodisks if they have rounded edges [20] . Both NSs and NPs have a thickness under 3 nm (1–2 atomic layers) [16] , [45] . Like 1D materials, 2D materials are also anisotropic, with tuneable properties, such as photothermal behaviour [46] , hydrophobicity [47] and stability in a range of chemical environments [48] , [49] , allowing 2D materials to be widely investigated for biomedical applications. Few-layered materials are formed when multiple atomic layers are stacked, and generally confined to a thickness of 3–50 nm thick, while their lateral area is typically under 1 cm 2 [27] , [49] . The antimicrobial mechanism of LDMs is multifaceted, with the precise mechanism of action varying between materials, systems and applications. This has important implications for the design, application and deployment of antimicrobial LDMs, and their use as viable treatments. To this end, it is important to classify the various modes of action to unlock their full potential as antimicrobial agents. Further, LDMs can be non-specific, meaning that potential synergistic or antagonistic effects must be assessed. Within existing literature, there is contention surrounding the antimicrobial mechanisms of LDMs. This is due to the complexity of the system as a whole, with interrelated and often simultaneous modes of action, the infancy of the field, and current experimental limitations often causing confusion [28] . As such, several mechanisms have been proposed, supported experimentally and theoretically, with both positive and negative correlations often being described. For clarity, we have assessed the currently reported LDM antimicrobial mechanisms and separated them into seven broad categories (Fig. 3 ). (1) Basal plane effects : Possessing a large surface area and amenability to chemical functionalisation, the basal plane of LDMs is believed to contribute to their antimicrobial activity. 2D materials have been observed to “wrap” microbial cells [50] , [51] , [52] , which is thought to inhibit nutrient/waste exchange [52] and/or cause perturbations in the integrity of the cell membrane through hydrophobic interactions [51] , [53] , or charge transfer effects [54] ; all cases resulting in cell lysis. The basal planes of 2D materials can also interact with intracellular lipids, proteins and nucleic acids, through π−π stacking, hydrogen bonding and electrostatic adsorption [28] . 0D [55] and 1D [56] , [57] nanomaterials have also been observed to demonstrate antimicrobial activity resulting from interactions with the basal plane. (2) Edge effects: The edge of LDMs possess unique physicochemical properties when compared to their respective bulk materials, which contribute to their antimicrobial action. Both 1D [56] , [58] and 2D [23] , [50] materials have been shown to puncture cell walls of microbial species upon contact, resulting in the leakage of intracellular components, and in-turn cell lysis. Experimental and theoretical studies demonstrate that 2D materials can translocate through the membrane in an orthogonal mode of penetration [59] , [60] , or form membrane-nanosheet sandwich structures [59] , [61] , due to different physico-chemical properties such as size and the degree of oxidation. These effects are not targeted and therefore, can pose a threat to mammalian cells. (3) Extraction of phospholipids from the membrane: Following an initial interaction with the edge of 2D materials, “nanoscale de-wetting” can occur due to strong hydrophobic interactions between the basal plane and the phospholipids, resulting in eventual membrane collapse [16] , [62] , [63] . Interestingly, 1D materials have been shown to exhibit similar phenomena on membrane models [64] however, studies on microbial cells have yet to be conducted. (4) Oxidative stress: Reactive oxygen species (ROS) can cause damage to important cellular components including proteins, nucleic acids and phospholipids, resulting in cell lysis [65] . ROS-independent oxidative stress can occur naturally in microbes, and interaction with or internalisation of LDMs can dramatically increase the intracellular ROS [66] . Conversely, LDMs can generate ROS in an aqueous media, which then interacts with the microbial cells [25] , [67] . For LDMs, the typically generated ROS species include singlet oxygen ( 1 O 2 ), superoxide anion radicals ( • O 2 – ), hydroxyl radicals ( • OH) and hydrogen peroxide (H 2 O 2 ). A summary of redox potentials for the generation of these ROS at physiological pH are shown in Supplementary Table 1 and referenced in Fig. 3 . (5) Light-driven mechanisms: This includes photocatalytic activity [31] , [68] , in which light, typically at a wavelength from ultraviolet (UV) to visible (Vis), drives the production of ROS which causes cell lysis. Alternatively, photothermal activity can be generated [25] , [46] , typically by light in the Vis-near infrared (NIR) wavelength region, which can cause a localised temperature increase which inactivates the microbial cells through membrane damage and the denaturation of enzymes [69] . (6) Synergistic effect: Combing LDMs can alter properties of materials, such as improved stability or enhanced antimicrobial activity [45] , [70] . One way the antimicrobial activity can be improved is in the form of releasing of ions or molecular species, also known as degradative effects [70] . Altering the materials properties, such as zeta potential, can promote new antimicrobial mechanisms [21] , [45] . (7) Other physical interactions: When 1D and 2D materials come into contact with microbial cells, they are able to physically damage the membrane [23] , [71] . This can be in the form of wrapping around, encapsulation or entrapping the cell, inducing cell lysis [56] . This is distinct from edge effects, which rely on either the electrical interaction of LDMs or physical damage, which occurs at the apex of an atomically sharp material. While these categories broadly cover the reported antimicrobial mechanisms of LDMs, these mechanisms often work simultaneously, and the relative importance of each is still debated. Broadly, the precise antimicrobial efficacy is likely to depend on: (1) biological factors, such as cell type, size and shape, (2) nanomaterial factors, such as size, shape and chemical functionality and (3) environmental factors, including, temperature, pH and components in the media such as proteins. Additionally, LDMs based nanocomposites have been developed which demonstrate multifaceted antimicrobial mechanisms and with enhanced treatment properties [6] , [70] . Fig. 3: Summary of the most accepted antimicrobial mechanisms of LDMs. A more detailed explanation of the mechanisms provided in antimicrobial mechanism section. Full size image The fabrication methodology of LDMs can also be used to manipulate their edges and basal planes. In general, synthesis of LDMs can be placed into two main categories: (1) bottom-up or (2) top-down methodologies. Bottom-up approaches are characterised by growing/synthesis from chemical precursors using a range of procedures and are more commonly used for metal oxides and 1D structures [72] , [73] . Alternatively, top-down synthesis occurs when a bulk material is broken down into the desired nanostructure and are typically used for 0D and 2D materials [25] , [74] . An effective and common method of utilising the antimicrobial properties of LDMs are as suspension-based approaches. LDMs can be suspended within a range of liquid medium and allow for the free movement of LDMs along with providing a possible environment for the generation of ROS. This section will highlight example LDMs in suspension with antimicrobial properties. Figure 4 shows common interactions of selected suspension-based LDMs and microbial cells to provide an overview for the reader. Fig. 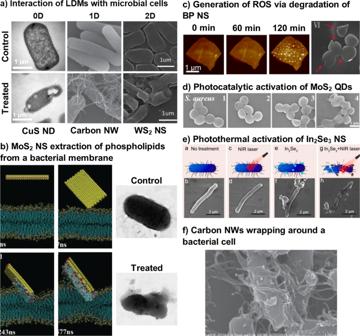Fig. 4: Summary of antimicrobial interactions of LDMs in suspensions. aInteraction of suspended Copper sulphide (CuS) NDs withEscherichia coli (E. coli)75, carbon NTs wrapping aroundLactobacillus acidophillus (L. acidophillus)56and tungsten disulphide (WS2) NSs withE. coli106.bThe extraction mechanism of membrane phospholipids by MoS2NSs63.cGeneration of ROS via degradation of BP NSs over 120 min (left)217and the interaction of Ti/BP NSs film withS. aureus(right) with cellular damage indicated with red arrows6.dPhotocatalytic activation of MoS2QDs against Staphylococcus aureus(S. aureus)74andethe photothermal activation of indium(III) selenide (In2Se3) NSs againstE. coli46.fCarbon NWs wrapping aroundL. acidophillus56. 4: Summary of antimicrobial interactions of LDMs in suspensions. a Interaction of suspended Copper sulphide (CuS) NDs with Escherichia coli (E. coli) [75] , carbon NTs wrapping around Lactobacillus acidophillus (L. acidophillus ) [56] and tungsten disulphide (WS 2 ) NSs with E . coli [106] . b The extraction mechanism of membrane phospholipids by MoS 2 NSs [63] . c Generation of ROS via degradation of BP NSs over 120 min (left) [217] and the interaction of Ti/BP NSs film with S. aureus (right) with cellular damage indicated with red arrows [6] . d Photocatalytic activation of MoS 2 QDs against S taphylococcus aureus ( S. aureus) [74] and e the photothermal activation of indium(III) selenide (In 2 Se 3 ) NSs against E. coli [46] . f Carbon NWs wrapping around L. acidophillus [56] . Full size image 0D materials Suspension-based 0D materials have several reported antimicrobial mechanisms, including cellular uptake [75] , radiation stimulus [74] and ROS generation [31] . Due to their innately small size, 0D materials can easily transverse microbial cell membranes, and enter the intracellular space (Fig. 4a ). This provides a unique capability to 0D materials, which is often not observed for 1D and 2D materials due to size constraints. Once inside the pathogenic cell, 0D materials can disrupt internal cellular processes (metabolic process, deoxyribonucleic acid (DNA) transcription, respiration, etc.) and also damage internal cellular material (DNA, ribosomes, and plasmids, etc.) [76] . The precise mechanism is dependent on the specific LDM, but 0D materials can rapidly lead to cell lysis following cellular uptake. Further, 0D materials have also shown potential for photo-induced antibacterial treatments (Fig. 4d, e ). Semiconductor QDs with a bandgap greater than 3.1 eV have demonstrated non-specific toxicity towards both mammalian and microbial cells when illuminated with UV light [72] . However, other semiconductor QDs are typically less toxic towards mammalian cells, hence more biocompatible, when excited under visible or NIR light [21] . Regarding the microbial toxicity, materials including carbon NDs (CDs) [77] , BP QDs [21] , cadmium telluride (CdTe) QDs [35] , MOs QDs [75] and MoS 2 QDs [74] , can generate excess ROS under visible, NIR and UV light irradiation. Metal oxides, such as ZnO QDs [78] , [79] and vanadium oxide (Vo x ) QDs [80] , [81] can also release ions under UV and ambient light irradiation. Tailoring the dimensions tunes the electronic structure of these LDMs to manipulate the wavelengths of light that activate the particles. Bare copper sulphide (CuS) QDs have three reported mechanisms, photothermal effects, Cu 2+ ion release and photodynamic generation of ROS under NIR [75] . These examples have demonstrated the importance of light in the antimicrobial mechanism of 0D materials, indicating the potential use in photodynamic therapy. Conjugating 0D materials with other LDMs can synergistically enhance the antibacterial mechanisms, by enhanced ROS production [78] or light assisted drug delivery [21] . Research into 0D materials as antimicrobial agents is relatively recent, and several materials have potentially favourable properties. BP QDs have recently been used for bioimaging and drug delivery applications, demonstrating biocompatiblility [82] . Larger TiO 2 NPs have demonstrated ROS generation, but research into QDs is lagging. While MXene QDs, including titanium nitride (Ti 2 N), Niobium carbide (Nb 2 C) and Ti 2 C 3 T x , have shown photothermal properties, with possible uses in cancer treatments and bioimaging [83] , to the best of our knowledge, no tests have been so far conducted into their potential use as antimicrobials. Further, bare WS 2 QDs had no antimicrobial impact, but when conjugated with antimicrobial peptides, it was effective against both Pseudomonas aeruginosa (P. aeruginosa ) and C. albicans biofilms [84] . This highlights the potential for more 0D materials to potentially have antimicrobial properties, or to have induced action through conjugation, but further exploration into these materials is needed. 1D materials Similarly, research into antimicrobial 1D structures, including carbon NTs [56] and a range of MOs [13] , [29] , is increasing. There are different antimicrobial mechanisms that have emerged in 1D materials (Fig. 4a ), such as carbon NTs, deactivate microbial cells through physical damage, which is heavily influenced by size [71] . For thinner single-walled NTs (SWNTs), the main mechanism is to puncture the bacterial membrane, acting as a nanodart/nanoknife [71] . Thicker, multi-walled NTs (MWNTs) tend to be less effective [71] and predominantly wrap around bacteria [56] (Fig. 4f ). Both SWNTs and MWNTs are potentially toxic against a range of microbes found in the human gut, including E. coli, S. aureus and Enterococcus faecalis (E. faecalis) [56] . Alternatively, MOs NRs and NWs mainly generate ROS to chemically induce cell lysis [85] . Interest into MOs has mainly focussed on ZnO [85] and CuO [86] , however recently other MOs, such as cerium(IV) oxide (CeO 2 ) [29] , magnesium oxide (MgO) [87] , maghemite (Fe 2 O 3 ) [88] and nickel(II) oxide (NiO) [40] , have demonstrated promising antimicrobial properties. ZnO materials can also release Zn 2+ ions, along with ROS, to aid in the damage of microbial cells [85] , indicating the possibility that LDMs with non-physical modes of action could have antimicrobial potential. There are several materials that have been shown to possess antimicrobial properties in their 2D form, but there is little research into their corresponding 1D forms. One material with such potential is graphitic carbon nitride (g-C 3 N 4 ), which generates ROS under light irradiation [89] . Recently, polymer functionalised BN NTs were also shown to have an increased efficacy compared to pristine BN NTs [90] . This further indicated how chemical modifications of 1D materials can enhance the antimicrobial activity to materials with little-to-no inherent efficiency. Other 1D materials have attracted interest for applications including gas sensing [18] , catalysis [91] and biomedicine [92] . Recent advancements in fabrication techniques have led to the synthesis of materials like BP NWs and NRis [18] , [93] , which to our knowledge have not been explored for their antimicrobial properties. 2D materials Recently, 2D materials have received considerable attention due to their relative ease of fabrication and their amenability to tuning their properties to make them responsive to a wider range of stimuli [45] , [48] , [94] . There are several common antimicrobial mechanisms observed in 2D materials, including physically slicing through the membrane [49] (Fig. 4a ), phospholipid extraction [62] (Fig. 4b ) or generating reactive oxide species [70] (Fig. 4c ). Graphene analogues Pure graphene has limited antimicrobial properties, while its oxide derivatives GO and reduced graphene oxide (rGO) have demonstrated broader antimicrobial capabilities [62] , [95] . Both GO and rGO can deactivate bacterial cells via oxidative stress [96] and piercing the membrane [53] , along with potential destructive extraction of the phospholipids comprising the membranes [62] . When GO was incorporated into an injectable hydrogel, its high photothermal properties and increased conductivity lead to improved antimicrobial activity against E. coli and MRSA [95] . It should be noted that the antimicrobial activity of graphene, GO and rGO remains controversial. A recent paper suggested that pure GO possess no inherent antibacterial character, but rather the widely reported behaviour is due to impurities [97] . Other graphene analogues also display antimicrobial properties. BP and hBN NFs have demonstrated the previously mentioned common antimicrobial mechanisms against E. coli and S. aureus [25] , [45] . Similar to GO, it has been speculated that hBN NSs cause membrane stress through lipid extraction [16] . BP NSs generate ROS under NIR light irradiation [25] , which can be enhanced when combined with larger nanoparticles [70] . Graphitic carbon nitride Another 2D carbon-based material with antimicrobial potential is g-C 3 N 4 . Pristine g-C 3 N 4 can effectively be used to treat against E. coli , MRSA and Bacillus anthracis spores, under visible or UV light irradiation conditions [98] . The functionalization of the g-C 3 N 4 surface using nitrogen plasma treatment (N-g-C 3 N 4 ) can increase the activity without requiring light activation [99] . The primary antimicrobial mechanism of pristine g-C 3 N 4 is via the photoactivated generation of free radicals [98] , while N-g-C 3 N 4 is thought to induce cell death mainly through the interaction with phospholipids within the cell membrane [99] . Metal oxides 2D MOs such as ZnO [94] , TiO 2 [12] , CuO [100] and MgO [27] have gained attention for effectiveness against a wide range of pathogenic microbes. The main antimicrobial mechanism used by MOs is the photo-induced generation of ROS [100] , [101] . 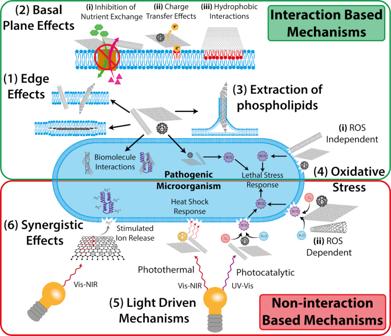Under visible light, MOs are effective treatments against S. aureus , E. coli and Staphylococcus epidermidis ( S. epidermidis) [27] , [102] , as well as under UV light [94] . Fig. 3: Summary of the most accepted antimicrobial mechanisms of LDMs. A more detailed explanation of the mechanisms provided in antimicrobial mechanism section. Some MOs including ZnO and CuO release cations that electrostatically disrupt the membrane [102] . Transition metal dichalcogenides TMDs also generate ROS and damage cellular membranes [49] . Recent studies have focused primarily on MoS 2 and WS 2 as potential antimicrobials as they are non-toxic [103] . The antimicrobial mechanism for MoS 2 is multifaceted, with the primary mechanism involving the generation of superoxide anions [67] , combined with slicing the membrane [49] and binding to peptide backbones [104] . Alternatively, WS 2 primarily deactivates cell through membrane damage, not through ROS [105] , [106] . The potential antimicrobial properties of other TMDs remain to be explored. Other 2D materials Several other 2D materials have shown potential for antimicrobial applications in limited studies but require further research. Preliminary studies into MXenes NSs, mainly Ti 3 C 2 T x , and indium(III) selenide (In 2 Se 3 ) have demonstrated activity against a limited number of Gram-positive and Gram-negative bacteria [24] , [46] , [50] . The sharp edges of the NSs play a key role in the degradation of the cellular membrane [24] . The photothermal properties of In 2 Se 3 can also be used to increase the antimicrobial efficacy [46] . As new LDMs are developed for use within other applications such as electronics or sensing, their potential as possible antimicrobial agents should be explored. Enhancing the antimicrobial capabilities of LDMs though heterostructuring will be discussed in a later section. Planar surfaces LDMs can be used to either generate or boost antimicrobial activity of a surface. For 1D and 2D materials, the orientation of the LDMs can influence the antimicrobial properties and affect the action of the primary antimicrobial mechanism (Fig. 5 ). The main orientations are vertical arrays [23] , horizontal coatings [107] or randomly oriented arrays [26] . These arrays and coatings can be used for implants [41] , wound dressings [15] , and other medically relevant surfaces [12] . Fig. 5: Summary of antimicrobial interactions with surfaces modified with LDMs. a Membrane damage of E. coli from TiO 2 NWs [8] and Cryptococcus neoformans from ZnO NWs (top and side view) [22] . b Various orientations of GO NSs on a surface and their interaction with E. coli [110] . c A multi-functional CuO NWs mesh with a superhydrophobic surface (left) which prevent E. coli and S. aureus growth (middle) and microbial adhesion after 5 days of incubation in domestic sewage water (right) [39] . Full size image Vertical arrays of LDMs are often reported for antimicrobial capabilities, through chemical activity and improved membrane damage, derived from their sharp edges (Fig. 5a, b ) [12] , [108] . 1D MOs have gained substantial attention as surface modifiers recently, with studies highlighting ZnO [22] , TiO 2 [12] and CuO [108] arrays as potential antibacterial and antibiofilm surfaces, as well as a possible antifungal treatment [22] . When MOs are grown in vertical arrays, there is a synergistic effect between the physical puncturing of the cellular membrane, the generation of ROS [22] , [108] , and the electrostatic interaction of the positive metal ions and the negatively charged membrane [109] . Combining 2D and 1D structures in an array can enhance photoactivated antibacterial properties by altering the electronic band structures of the materials. When rGO NSs are combined with CuO NWs, the CuO injects an electron into the rGO, allowing for enhanced ROS generation under visible light irradiation [108] . A recent study found that a higher edge density of an array can improve the antimicrobial activity, whilst also supressing any mechanisms of the substrate, such as wrapping [23] . The morphology of the LDMs in the vertical array influences the antimicrobial efficacy; however, more research is needed to identify they key parameters for optimisation. Similarly, randomly orientated LDMs (Fig. 5b ) are used to enhance the antimicrobial properties of a surface. These materials are still able to penetrate cellular membranes through edge effects; however, the number of edges in the preferential orientation is reduced [26] , [110] . Randomly orientated GO NSs effectively reduced a population of E. coli by 25%, compared to 44% for vertically aligned NSs [110] . Although the main mechanism for GO NSs is still being investigated, the decreased efficacy of random NSs was attributed to the decreased penetration of the cellular membrane [110] . Randomly orientated 1D MOs NWs can influence the hydrophobicity of the surface, leading to a two-stage mechanism (Fig. 5c ). The more tightly packed surfaces increase the hydrophobicity, preventing cellular adhesion. Once cells begin to settle, the NWs can puncture the membrane, whilst the chemical activity of the MOs NWs also provide longer-term antimicrobial action [26] . Initial research has been conducted into the relationship between material angle, microbial adhesion and membrane penetration. As fabrication methods continue to advance to allow for greater control of the angle, this relationship can be explored in more detail to allow for greater optimisation. Although still capable of antimicrobial action, horizontal or planar LDMs (Fig. 5b ) are not as effective as the previously mentioned orientations. When deposited horizontally, LDMs are more reliant on chemical mechanisms, as the physical antimicrobial mechanisms derived from edge effects are limited [15] , [110] . For 1D MOs deposited horizontally, electrostatic interactions of ROS are predominantly used to inactivate cells [15] , [41] . In the case of CeO 2 NRos deposited onto medical-grade titanium, the material was able to reduce biofilm formation of common plaque-forming bacteria by 99%. The main antimicrobial mechanism is believed to be via electrostatic interactions between the CeO 2 NRos and the cell membrane [41] . Horizontally orientated TiO 2 NWs coatings rely on ROS, as the NWs are more efficient at photodegradation than larger nanoparticles [15] . Horizontally deposited NSs tend to show lower antimicrobial activity compared to vertically orientated NSs [107] , [110] . For example, horizontal GO NSs resulted in a ~20% reduction of E. coli cells, in comparison to 44% for the vertical GO NSs [110] . MoS 2 NSs have been shown to reduce E. coli growth by roughly 50% after a 3 hour incubation [107] . Surfaces can also be modified with the addition of 0D materials to improve their antimicrobial properties. The antimicrobial activity of 0D material modified surfaces has been investigated across a broad range of medically relevant materials, such as wound dressings [111] , [112] , resins [113] , polymers [114] and drug delivery systems [115] . Due to the shape of 0D materials, chemical pathways such as ROS generation [112] or electrostatic interactions [115] are the main antimicrobial mechanism. Depositing carbon and graphene QDs onto common fabric bandages prevent E. coli and S. aureus growth and promoted wound healing via photo-induced ROS [112] . When carbon QDs were doped with nitrogen, they were capable of treating MRSA infections to the same degree as the antibacterial drug vancomycin [111] , indicating its potential use in treating vancomycin-resistant Enterococcus infections. Biofilm formation of Streptococcus mutans , a common dental pathogen, had a 99% reduction after exposure to an adhesive dental resin coated with ZnO QDs [113] . Further, E. coli and S. aureus growth was reduced by ZnO QDs deposited onto bioactive glass nanoparticles [79] . The antimicrobial action of 0D materials can be increased by depositing multiple materials that have a combined effect. The ROS generation of ZnO can be increased by also depositing cadmium sulphide (CdS) QDs onto the surface and activating using UV light. Combining both QDs with the polysaccharide chitosan prevented both E. coli and Bacillus subtilis ( B. subtilis) growth [115] . Using 0D materials as additives in materials with inherent antimicrobial properties can also increase the effectiveness. Under ambient light, indium-based QDs were not effective against clinical and environmental strains of P. aeruginosa and E. coli . Combing the indium-based QDs with crystal violet increases light absorbance and increases ROS generation to a lethal amount [114] . Three-dimensional filters LDMs can be deployed to improve water filtration to prevent infections from waterborne pathogens. One method to increase the efficacy of water filtration is to increase the hydrophilicity of the filter. This can be achieved by depositing 2D materials such as WS 2 [48] or g-C 2 N 4 [116] , [117] , or growing 1D materials like Cu NWs [39] (Fig. 5c ). WS 2 was able to reduce the amount of E. coli and S. aureus in solution by around 90% [48] . Photocatalytic materials such as g-C 2 N 4 NSs also generate ROS under visible light exposure and have been shown to cause an over 99.99% reduction E. coli from solution [117] . Cu NW mesh uses multiple antimicrobial mechanisms, including super hydrophilicity, the generation of Cu + ions and photothermal interactions [39] . MXene membranes have also demonstrated antifouling properties and were effective against both E. coli and B. subtilis via oxidation and photothermal reactions [118] . Another application for LDMs is enhanced filters for use in air purification to reduce the spread of airborne pathogens. Fe 2 O 3 NWs grown on an iron mesh to capture common indoor bioaerosols via the generation of hydroxyl radicals [73] . A single filter was able to capture 52% of airborne S. epidermidis and E. coli , and 5 filters in tandem were able to reduce airborne cells by 98%. Although a promising application, the instability of several LDMs in ambient conditions has limited their potential to be used for air purification. When dissimilar materials are stacked in layers, they can result in new properties which have typically been used to great effect in electronics and optoelectronics [119] , [120] . The ability to stack materials of desired size/thickness and different phases (solid/liquid) in lateral or vertical heterostructures, allows the manipulation of physical and electronic properties of the material at the atomic scale via quantum engineering [121] . The use of LDMs can be considered a win–win solution in the quest for achieving a combination of antimicrobial properties. Combining materials can aid in passivating materials from ambient degradation that otherwise show outstanding antimicrobial properties. These hybrid materials can also be prepared in a solution phase which can be used as surface/spray coatings on the implants using the dispersion technology [122] . The materials used to form heterostructures are usually chosen from the periodic table among the III-V, IV-IVI, II-VI groups. The material systems are stacked, altering their band structures to benefit the desired applications [119] (See supplementary document). Recent advancements in LDMs have highlighted their potential as antimicrobial treatments. These highly antimicrobial materials can reduce the number of microbial cells by over 80% within a few hours. Such materials include: (1) 0D [77] and 1D [71] carbon, (2) 0D [123] and 2D [124] g-C3N4, (3) 0D CdTe [35] , (4) 1D metal oxides [29] , [109] , (5) 2D GO [110] , (6) 2D BP [41] , [70] and (7) 2D MXene [24] , [50] , which have all exhibited high antimicrobial ability. Most of these materials employ a combination of mechanisms that are influenced by their chemical composition and morphology [27] , [117] . There are many factors to consider when selecting LDMs for a specific antimicrobial treatment or scenario. For instance, is the desired application biological or abiotic in nature? What is the delivery method of the required treatment (injectable, solution, surface, physical, etc)? Does the treatment need to last for a prolonged period, or does it degrade rapidly in response to treatment? Is there a single target pathogen or more-general antimicrobial activity required? Is a chemical approach or physical methodology better for the scenario in question? To assist with answering these questions, the following section has been designed to give an overview of the currently available antimicrobial LDMs and provide insight into the future directions of research in this area. 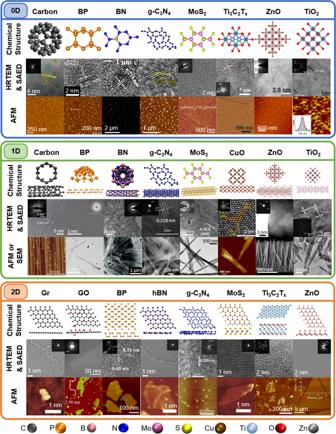Notably, the selection of LDMs is not trivial and is dependent on the system, application and specific microbes involved. Furthermore, the application must be adequately tailored to either prevention or treatment. Fig. 2: Visual summary of common LDMs. 0DThe chemical structure (top), high-resolution transmission electron microscope (HRTEM) image (inset is corresponding selected area electron diffraction (SAED) pattern where applicable) (middle) and atomic force microscopy (AFM) scan (bottom) for carbon dots77,200, BP QDs201, BN QDs202, g-C3N4 QDs123, MoS2NDs168, Ti3C2TxQDs83, ZnO QDs133,203and TiO2QDs129,204.1DThe chemical structure (top), HRTEM image (inset is corresponding SAED pattern) (middle) and AFM scan or scanning electron microscope (SEM) image (bottom) for carbon NWs205, BP NWs18, BN NFs206/NTs207, g-C3N4NRs179,208, MoS2NWs91,209, CuO NRs86, ZnO NWs22,210and TiO2NWs12/NTs211.2DThe chemical structure (top), HRTEM image (inset is corresponding SAED pattern) (middle) and AFM scan (bottom) for graphene (Gr) NSs192, GO NSs212,213, BP NSs194, hBN NSs192, g-C3N4NSs214, MoS2NSs192, Ti3C2TxNSs43,215and ZnO NSs216. Table 2 summarises the currently measured antimicrobial efficacy, the respective cytotoxicity, relative commercial costs, chemical stability, and the current status of the LDMs previously described for medical, industrial, and scientific-based antimicrobial-based exploitation. Table 2 Summary of LDMs for antimicrobial applications [218] , [219] , [220] , [221] , [222] , [223] , [224] , [225] , [226] , [227] , [228] , [229] , [230] , [231] , [232] , [233] , [234] , [235] , [236] , [237] , [238] , [239] , [240] , [241] , [242] , [243] , [244] , [245] , [246] , [247] , [248] , [249] , [250] , [251] , [252] , [253] , [254] , [255] , [256] , [257] , [258] , [259] , [260] , [261] , [262] , [263] . Full size table When considering using LDMs within a biological system, the biocompatibility with mammalian cells is an essential factor. Table 2 summarises which LDMs have been tested for their effect on mammalian cells, either using cell cultures (in vitro) for 48–72 h [41] , [125] or live mouse models (in vivo) for over a period of seven days [81] , [126] . If the material has demonstrated non-selective toxicity towards both microbial and mammalian cells, their use in treatment is not desirable. Utilising the chemical routes for antimicrobial activity Many LDMs that have demonstrated high antimicrobial activity can generate ROS. The ability to generate ROS in solution is directly linked to LDMs bandgaps and therefore redox potentials, with the bandgaps of numerous LDMs discussed above falling into the range 1.5–3.5 eV (see Table 1 ). These bandgaps are sufficient to elicit the generation of ROS (Supplementary Table 1 ) in solution, which can damage the microbial cell wall. Therefore, if the antimicrobial action requires the production of ROS, the use of materials which fall outside of this range is not recommended. LDMs that have demonstrated antimicrobial activity and are capable of generating ROS species in solution include BP [70] , MXene [118] and WS 2 [103] . However, there are also LDMs that do not generate ROS, but is still possess antimicrobial activity such as 2D hBN [127] , which has limited antibacterial efficiency [90] , [128] . For such materials, forming composites or heterostructures can alter their intrinsic bandgaps, and facilitate the generation of ROS [115] , [129] . In some systems, the generation of ROS can be promoted via the addition of ultra-low concentrations of hydrogen peroxide [81] , [112] . LDMs which readily degrade into fragments, ions, sub-species and/or ROS can be advantageous for antimicrobial treatments or surface-functionalisation. For example, BP is well known to degrade under ambient atmosphere and solution conditions, producing ROS and P x ions [130] , [131] . The ability for the material to both degrade and produce antimicrobial species is useful for applications which require the biocidal agent to disintegrate from the treatment zone without removal. Other LDMs degrade at a slower rate, such as In 2 Se 3 , and have also shown potential antimicrobial activity [132] . This degradation or generation of ROS can also be enhanced using light irradiation [35] , [124] . LDMs that have demonstrated photocatalytic properties can potentially be used to assist with targeted treatments [21] . Morphological and physical exploitation The morphology, size, surface charge and flexibility of LDMs can positively and negatively correlate to biocidal enhancement in both suspension-based and surface-based technologies. Broadly, the degree of antimicrobial activity within a system is both species and treatment dependent and represents an interplay between contributing factors. However, the precise nature of the LDM-microbial interactions is still relatively poorly understood, often resulting in conflicting results, even amongst similar systems. The following section aims to collate the current level of understanding of the morphological and physicochemical interactions which facilitate LDM antimicrobial action. For 0D materials, cellular uptake, electrostatic disruption, and specific cell–surface interactions are the primary physical modes of action. Here, the comparatively small size of the material facilitates cellular uptake, which is often not achieved by larger 1D and 2D materials. This means that the physical size and surface chemistry of the material is a key determining factor. If an application requires intracellular interactions, then 0D materials are prime antimicrobial candidates - smaller 0D LDMs can possess enhanced activity [133] . Further, 0D materials are known to facilitate intra- and extracellular damage via unfavourable electrostatic interactions. However, we found no reports of 0D LDMs that cause physical-based membrane rupture. For 1D and 2D materials, the aspect ratio can influence the antimicrobial activity [29] . For CeO 2 NRs, a higher aspect ratio resulted in more active sites on the NR surface, generating a higher concentration of hypobromous acid (HOBr), increasing the antimicrobial activity [29] . The aspect ratio can also be linked to the cytotoxicity of a material [29] . For some materials, a higher aspect ratio increases the toxicity towards human cells [29] . 1D CuO NW mesh was found to be superhydrophobic and prevented bacterial adhesion [39] . For 2D sheets, the edges of the material are known to be “sharp” and induce microbial cells damage upon cell-on-edge adsorption. Several forces are at play when LDMs and microbes interact, including electrostatic, van der Waals and hydrophobic forces. Together, these forces can lead to microbial membrane damage during LDM material interactions. It should be noted that LDM-pathogen interactions are complex, possessing contributions from both the material and the microbial cell. For instance, the surface chemistry, charge, hydrophobicity, inherent roughness, geometry and free energy are all contributing factors from the LDM material. For the pathogen, molecular composition, surface charge, hydrophobicity, extracellular polymeric substance (EPS) and cell appendage interactions all play a role. In general, it has been suggested that positively charged materials attach to the negatively charged microbial membrane to induce membrane damage [45] , [100] . Some materials can deactivate membrane components, such as the thiol group, through the generation of ions [41] , [100] or by extracting of phospholipids [62] , [63] . Ions are typically generated by MOs, which cause the leakage of intracellular components [39] , [79] or directly damage the intracellular components [134] . Pre-infection treatments One application for LDMs is in preventing microbial infections (i.e. pre-infection treatment) via limiting microbial adhesion to surfaces [26] , [135] and decreasing microbial growth [32] , [79] . For LDMs to be used as an effective pre-infection treatment, they will need to be in a portable form with long-term stability, such as a bandage or implant coating or LDMs suspended in hydrogel [95] , [112] . External stimuli can be applied to prevent infections in a clinical setting but are not practical for consumer products. Similarly, the chemical stability of LDMs must be improved for commercial products as they will need to be stored for longer periods. Overall antimicrobial activity is another important property to consider when using LDMs for pre-infection treatments. Materials, such as BP NSs [45] and g-C 3 N 4 QDs [123] , can be used as fast-acting treatments, while other materials including 0D MOs [41] , [136] and MXene NSs [137] have shown antimicrobial activity over several days. This duration is important as it influences the frequency of treatments, and how often the wound is exposed to unsterile conditions, increasing the risk of re-infection. Post-infection treatments Once an infection has formed, it can become much harder to treat and prevent more entrenched infection [138] , [139] . The use of stimuli-activated LDMs, such as photothermal [75] or photoactivation [35] could be utilised within clinical settings. Importantly, LDMs have the ability to treat established infections with large quantities of microbial cells [138] , [140] . One method of achieving this higher microbial inactivation can be the use of external stimuli, such as light activation [123] , [141] . Several materials, including 1D MOs [26] , [41] , [140] and graphene QDs [112] have been able to reduce pre-existing biofilms by over 90% following photoactivation. Following the initial treatment to reduce the infection, previously discussed pre-infection treatments can be used in tandem to help prevent another infection. Computational modelling as a guide for future treatments Computational modelling techniques have demonstrated great potential to aid in the understanding of existing antimicrobial mechanisms and guide development of new LDMs. Classical molecular dynamics (MD) simulations have been used to show in atomistic detail how GO, N-g-C 3 N 4 and MoS 2 nanosheets can destructively extract lipids from bacterial membranes [62] , [63] , [99] (Fig. 6a ). In addition, coarse-grained MD simulations allow for a direct and fast in silico screening of LDMs candidate materials [142] . MD simulations have also shown why some LDMs are effective in vitro but not in vivo. For example, Duan et al. demonstrated that the efficacy of GO as an antimicrobial agent was significantly reduced by the presence of a protein corona formed by serum proteins that reduced the available surface area and sterically hindered membrane penetration and disruption [143] . On the other hand, MD simulations have also shown how the effects of a protein corona can be overcome, or even utilised advantageously, for cell penetration of functionalized nanoparticles [144] . While MD simulations are useful for studying interactions that can occur between LDMs and microbial membranes or biofilms [145] , [146] , quantum chemical (QC) methods can calculate bandgaps of candidate LDMs [147] , [148] , or examine the reaction mechanisms involved in ROS generation. Taking BP as an example, while the full ROS production reaction mechanism has yet to be elucidated, studies have shown that initial reactions leading to ROS production and BP degradation are most likely to occur at edges and defects in BP [17] , [149] (Fig. 6b ). For the rapid and efficient exploration of a large number of candidate LDM properties, machine learning (ML) is often the best approach. ML algorithms can predict properties ranging from bandgaps of MXenes and hybrid 2D materials [150] , [151] to biocompatibility of ZnO nanoparticles [152] . Fig. 6: Atomistic modelling of antimicrobial LDM behaviour. a Lipid extraction by graphene oxide nanosheets from the outer membrane surface [62] . b Top view and side view of the reaction of O 2 (red) with monovalent defect BP (purple) from QC calculations. Full size image LDMs with little or no antimicrobial activity Although many LDMs have demonstrated high antimicrobial efficiency (over 80% cell death within several hours), there are some materials with little or no antimicrobial action. These materials were only capable of killing less than 60% of the microbial cells in 3 h or required over 8 h to inactive over 70% of microbial cells. These materials include hBN NSs [153] , WS 2 QDs [84] , BP QDs [21] and graphene NSs [154] . Some morphologies of these materials have demonstrated higher antimicrobial efficiency. One example of decreased antimicrobial action is BP, with the 2D BP achieving over 80% cell death within an hour [25] , [70] , compared to QDs, which reached 60% cell death after 2 h [21] . Another example of a material with little antimicrobial activity is 2D hBN, with a 30% cell reduction in 3 h [153] . This reduced antimicrobial activity is likely due to hBN not generating ROS, which means it is more reliant on a physical rather than a chemical mechanism which limits the overall antimicrobial potential [127] , [153] . A careful review of the literature reveals the several QDs have lower antimicrobial activity compared to their 1D or 2D counterparts. This may be due to their antimicrobial activity arising from chemical/ion interactions [74] , [79] , while having diminished ability to induce membrane damage. The medium of the LDMs can also influence the antimicrobial efficiency. MOs have an increased antimicrobial potential on a surface [12] , [140] , where most 0D materials are more effective as a suspension [72] , [77] . For LDMs that rely on chemical interaction, suspension-based approaches have a higher antimicrobial efficiency [72] , [140] . In contrast, physical-based antimicrobial mechanisms are efficient as both surface- and suspension-based treatments, depending on the desired application [23] , [116] . For water purification, membranes equipped with LDMs are more effective than LDMs freely suspended in solution, and do not have to be removed from the purified water [27] , [39] . For wound treatments, however, depositing LDMs onto traditional wound dressing surfaces, such as bandages or adhesive resins, have shown to promote improved wound healing compared to untreated dressings [75] , [112] . Although LDMs have promising antimicrobial properties, there are still limitations in fabrication processes and scalability that prevents practical implementation, for instance; 1. Synthesis methods for LDMs often use toxic solvents [87] , [137] , require prolonged synthesis at high temperatures [18] , [116] and result in low yields [25] , [111] . 2. Many 1D nanostructures, aside from MOs and GO, have only recently been synthesised and currently lack exploration into possible antimicrobial activity [18] , [93] . 3. Some LDMs are less stable in desired environments such as in air or in solutions with a neutral pH [25] , [136] . One of the significant concerns using LDMs within a medical and commercial setting are related to their fabrication. Although LDMs should be available for feasible consumer products, consistent, cost-efficient methods need to be developed to allow for batch production. Major challenges to resolve for LDMs to attain market growth include (1) scalability, especially roll-to-roll manufacturing, (2) repeatable and reliable fabrication methods, (3) low contact resistance and (4) LDM-based precise characterisation techniques. One key point to a favourable outcome is the capability to prepare 2D materials at the wafer level. In this way, it will be possible to create large amounts of 2D devices for fabrication and decrease product cost [120] . The current use of either high temperatures or toxic solvents [18] , [116] has led to an increased interest in developing green synthesis routes using natural materials for LDMs fabrication [40] , [82] , increasing the potential for wider biomedical applications. Several current fabrication processes can take several days [15] , [47] , and long-term storage can be limited [24] , [49] . One method of overcoming the rapid degradation of LDMs is to suspend the LDMs in liquid stabilisers or through storage in controlled environments [35] , [136] . For example, some materials require a specific pH for storage of more than a few weeks, which is not ideal for biomedical applications [35] , [72] . Although these stabilising measures are effective within a controlled laboratory setting, implementation on a larger scale for practical use is limited. For clinical applications, stabilisation could be achieved by embedding LDMs in medically relevant materials currently being used as wound treatments, such as hydrogels [155] . The scalability and long-term impacts of LDMs on biological systems still require more research. There have been some cytotoxicity studies for a range of LDMs but these are predominantly carried out using in vitro cell cultures or mouse models [81] , [125] . However, the method of excretion of LDMs from vital organs and the potential risks posed by LDMs aggregating within the body still needs to be examined futher [109] , [125] . Within the published literature, most LDMs have only been tested against a few key bacterial strains. The most common models are S. aureus for Gram-positive and E. coli for Gram-negative bacteria, which are human pathogens capable of significant morbidity and have several documented drug-resistant strains [48] , [79] . Often in biological studies, fungal cells are overlooked, even though they pose a similar health threat [5] . This is important as fungal cells are larger than bacteria cells and possess different membrane structures and hence can be impacted differently by the antimicrobial mechanisms generated by LDMs [22] . 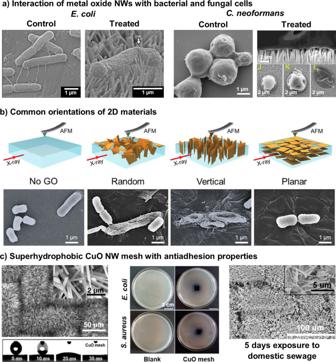Fig. 5: Summary of antimicrobial interactions with surfaces modified with LDMs. aMembrane damage ofE. colifrom TiO2NWs8andCryptococcus neoformansfrom ZnO NWs (top and side view)22.bVarious orientations of GO NSs on a surface and their interaction withE. coli110.cA multi-functional CuO NWs mesh with a superhydrophobic surface (left) which preventE. coliandS. aureusgrowth (middle) and microbial adhesion after 5 days of incubation in domestic sewage water (right)39. 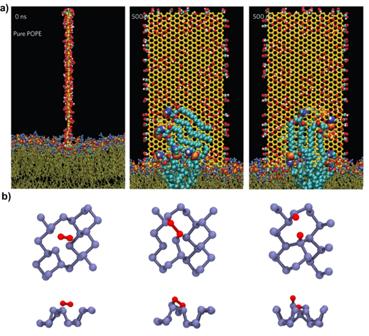Fig. 6: Atomistic modelling of antimicrobial LDM behaviour. aLipid extraction by graphene oxide nanosheets from the outer membrane surface62.bTop view and side view of the reaction of O2(red) with monovalent defect BP (purple) from QC calculations. Another limitation of the current microbial testing is the lack of “real world” scenarios. For example, if biofilm prevention is tested, typically only single strain models are used with limited testing on biofilms containing multiple bacterial strains, which are common on implant-associated infections [12] . LDMs [1] , [35] , [45] , [156] utilise a combination of chemical and physical modes of action to kill pathogenic microbes with extremely high efficacy in a range of conditions. Combining this with the emerging capability to control the properties of LDMs offers an unprecedented opportunity for the research community to explore a plethora of potential antimicrobial applications. Furthermore, the synthesis of composites LDMs which can have synergistic effects provides the basis to create new paradigms in a field of antimicrobials, which has stagnated to a dangerous point [24] , [71] . Importantly, there is a lot more work that needs to be done. Many facets of the antimicrobial mechanisms of LDMs remain unclear, and the library of prospective materials should be expanded. Further, the clinical and commercial applications of these materials remain under researched. Such areas of research need to be further investigated for LDMs to be considered a serious alternative to current antimicrobial treatment strategies. It is hoped that this review will provide a foundation for informed decisions and design parameters of next-generation antimicrobial LDMs with antipathogenic activity and reveal an antipathogenic technology capable of combatting AMR pathogens.